Tumour angiogenesis regulation by the miR-200 family The miR-200 family is well known to inhibit the epithelial–mesenchymal transition, suggesting it may therapeutically inhibit metastatic biology. However, conflicting reports regarding the role of miR-200 in suppressing or promoting metastasis in different cancer types have left unanswered questions. Here we demonstrate a difference in clinical outcome based on miR-200’s role in blocking tumour angiogenesis. We demonstrate that miR-200 inhibits angiogenesis through direct and indirect mechanisms by targeting interleukin-8 and CXCL1 secreted by the tumour endothelial and cancer cells. Using several experimental models, we demonstrate the therapeutic potential of miR-200 delivery in ovarian, lung, renal and basal-like breast cancers by inhibiting angiogenesis. Delivery of miR-200 members into the tumour endothelium resulted in marked reductions in metastasis and angiogenesis, and induced vascular normalization. The role of miR-200 in blocking cancer angiogenesis in a cancer-dependent context defines its utility as a potential therapeutic agent. The miR-200 family has been shown to potently inhibit the epithelial–mesenchymal transition (EMT) by downregulating ZEB1 and ZEB2 . The ability to reverse this process has been repeatedly demonstrated in vitro with miR-200 restoration [1] , [2] , [3] . Surprisingly, however, although forced miR-200 expression can inhibit the formation of distant metastasis in lung cancer, it can enhance metastasis in breast cancer models [4] , [5] . The latter effect appears to be driven, in part, through miR-200-mediated downregulation of Sec23a (ref. 4 ). Other studies suggest the existence of differences in the effects of miR-200 expression on clinical outcome [4] , [6] , [7] , [8] , [9] , but most of these are limited by small sample sizes, heterogeneous subtypes and different statistical methods. These observations prompted us to consider potential mechanistic differences based on cancer type that would explain differences in miR-200-driven biology. Here we have uncovered previously unknown mechanisms and context behind miR-200’s role in regulating cancer progression. We demonstrate that in ovarian, lung, renal and basal-like breast adenocarcinomas, elevated miR-200 expression portends improved clinical outcome, in part, through the regulation of angiogenesis by inhibiting key pro-angiogenic cytokines (interleukin (IL)-8 and CXCL1). As such, these findings have implications for personalizing miR-200-based therapy. Clinical outcomes of miR-200 expression vary across cancers Using the Cancer Genome Atlas (TCGA) data, we first chose to analyse four adenocarcinomas (ovarian, lung, renal and breast) with clinically annotated samples ( Supplementary Data 1 ). Expression data for all five miR-200 family members (miR-141, -200a, -200b, -200c and -429) were obtained. In training and validation cohorts, for ovarian ( n =579; P =0.019, log-rank test, Fig. 1a ) and renal cancers ( n =474; P =0.005, log-rank test, Fig. 1a ), low expression of a miR-200 family member was significantly associated with worse overall survival. In lung adenocarcinomas, low expression of several miR-200 isoforms was significantly associated with worse overall survival ( Supplementary Fig. S1a ). However, in breast cancer ( n =325), low expression of a miR-200 member was associated with improved clinical outcome ( P =0.036, log-rank test, Fig. 1a ). Consistent with these observations, multiple other miR-200 members for each tumour type were significantly associated with clinical outcome ( Supplementary Table S1 ). Of note, the worsened survival in breast cancer was only significant for the luminal subtypes ( Supplementary Fig. S1b ), suggesting miR-200 may have unique gene regulation across the different breast cancer subtypes. Because of high associated mortality and a possible role for miR-200b in lung adenocarcinoma [9] , [10] , we further assessed the significance of miR-200b expression using in-situ hybridization in a separate cohort of 121 non-small cell lung cancer patients. Consistent with our findings from TCGA, low miR-200b was significantly associated with worse overall survival ( P =0.029, log-rank test, Fig. 1b ), especially in lung adenocarcinoma ( P <0.0001, log-rank test). 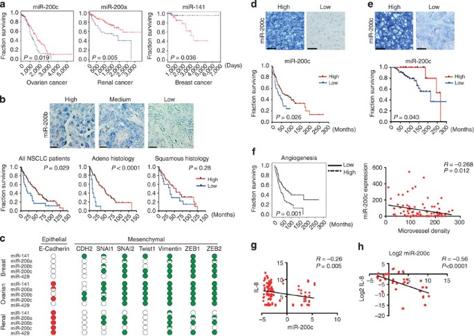Figure 1: Divergent clinical outcomes and network regulation by the miR-200 family. Kaplan–Meier curves for overall survival for high and low expression of miR-200c in ovarian cancer, miR-200a in renal cancer and miR-141 in breast cancer (a). (Blue, low expression; red, high expression.) (b) miR-200b expression levels (in-situhybridization) in non-small cell lung cancer (NSCLC). (Top) Representative images of high, medium and low expression, and (bottom) Kaplan–Meier curves for overall survival for high and low expression in all lung samples (left,n=121), adenocarcinomas (middle,n=69) and squamous cell carcinomas (right,n=52). Scale bars, 250 μm. (c) Student’st-test comparison of the expression levels of epithelial and mesenchymal markers in breast, ovarian and renal samples above and below the median miR-200 expression levels. (Green, increased expression; red, decreased expression; non-filled dots, not significant; half-filled dots,P<0.05; filled dots,P<0.01, Student’st-test.) Kaplan–Meier curves for overall survival based on miR-200c expression (in-situhybridization, representative high and low expression are shown) in serous ovarian carcinoma (n=160) (d) and basal-like breast cancers (n=103) (e). Kaplan–Meier curves for (f) microvessel density (left) in ovarian cancer. Pearson’s correlation for miR-200c and (f) microvessel density (right). Scale bars, 250 μm (b–e). (g) Pearson’s correlations for microarray expression levels from the NCI-60 cell line panel for IL-8 versus miR-200c. (h) Spearman’s correlation of miR-200c and IL-8 expression levels of a 27 cell line panel. Figure 1: Divergent clinical outcomes and network regulation by the miR-200 family. Kaplan–Meier curves for overall survival for high and low expression of miR-200c in ovarian cancer, miR-200a in renal cancer and miR-141 in breast cancer ( a ). (Blue, low expression; red, high expression.) ( b ) miR-200b expression levels ( in-situ hybridization) in non-small cell lung cancer (NSCLC). (Top) Representative images of high, medium and low expression, and (bottom) Kaplan–Meier curves for overall survival for high and low expression in all lung samples (left, n =121), adenocarcinomas (middle, n =69) and squamous cell carcinomas (right, n =52). Scale bars, 250 μm. ( c ) Student’s t -test comparison of the expression levels of epithelial and mesenchymal markers in breast, ovarian and renal samples above and below the median miR-200 expression levels. (Green, increased expression; red, decreased expression; non-filled dots, not significant; half-filled dots, P <0.05; filled dots, P <0.01, Student’s t -test.) Kaplan–Meier curves for overall survival based on miR-200c expression ( in-situ hybridization, representative high and low expression are shown) in serous ovarian carcinoma ( n =160) ( d ) and basal-like breast cancers ( n =103) ( e ). Kaplan–Meier curves for ( f ) microvessel density (left) in ovarian cancer. Pearson’s correlation for miR-200c and ( f ) microvessel density (right). Scale bars, 250 μm ( b – e ). ( g ) Pearson’s correlations for microarray expression levels from the NCI-60 cell line panel for IL-8 versus miR-200c. ( h ) Spearman’s correlation of miR-200c and IL-8 expression levels of a 27 cell line panel. Full size image Unique miR-200-regulated networks based on cancer type Next, we performed integrated network analyses to investigate possible mechanisms of divergent clinical outcomes based on miR-200 expression. Although in breast, renal and ovarian cancers, nearly all of the mesenchymal markers were downregulated in the high miR-141, miR-200a and miR-200c expression subsets, respectively, E-cadherin was significantly upregulated only in ovarian and renal cancers ( Supplementary Table S2 ). We also tested potential associations between the five miR-200 members and EMT genes. For each miRNA, the samples were divided into two groups consisting of high or low miRNA expression. As before, mesenchymal markers were significantly downregulated in the high miR-200 expression subset for breast, renal and ovarian cancers; however, E-cadherin was significantly upregulated only in ovarian and renal cancers ( Fig. 1c , Supplementary Table S3 ). Furthermore, E-cadherin was not significantly increased in basal-like or luminal breast cancer subtypes based on miR-200 member expression ( Supplementary Table S4 ). In addition, in basal-like or luminal breast cancer cell lines, E-cadherin was not consistently increased following transfection with miR-200 members ( Supplementary Fig. S2 ). Surprisingly, regardless of the threshold chosen in ovarian and renal cancers, E-cadherin was not significantly associated with overall survival, indicating that miR-200’s clinical relevance is likely linked to the regulation of other key networks. To examine potential differences in signalling networks across miR-200 members, we first identified all genes that were significantly inversely correlated with each miR-200 member. Then, from this initial gene set we used predictive software analysis to enrich for genes that may be regulated by miR-200. A pathway analysis was then performed to test for association with key signalling networks. For breast cancer, an integrated network analysis for each subtype (for example, luminal, Her-2 and basal-like) was performed using the TCGA data [11] ; miR-200 significantly regulated DNA-dependent transcription regulation ( P =3.4 × 10 −9 , Benjamini–Hochberg multiple testing correction) and metabolic processes ( P =4.6 × 10 −8 , Benjamini–Hochberg multiple testing correction) in luminal type; whereas in Her-2 subtypes, cytoskeletal protein binding ( P =3.6 × 10 −4 , Benjamini–Hochberg multiple testing correction) was the most significantly regulated network ( Supplementary Fig. S3a ). However, in basal-like breast cancers, some of the most significant miR-200 networks regulated were related to angiogenesis ( Supplementary Fig. S3a ). Similar findings were noted in high-grade serous ovarian cancers ( P <1 × 10 −6 , Benjamini–Hochberg multiple testing correction, Supplementary Fig. S3b ) known to have substantial molecular similarities with basal-like breast cancer [11] , and for renal and lung adenocarcinomas ( P =2 × 10 −3 for renal, P =3 × 10 −3 for lung, Benjamini–Hochberg multiple testing correction; Supplementary Fig. S3c,d ). Next, on the basis of pathway analyses described above, we determined whether the expression of miR-200 members correlated with survival using separate cohort of ovarian and breast cancer samples. Similar to our findings from the TCGA analysis, decreased miR-200c expression was associated with significantly worse overall survival in ovarian ( P =0.026, log-rank test, Fig. 1d ) and basal-like breast cancer ( P =0.043, log-rank test, Fig. 1e ). Positive and negative hybridization controls are provided in Supplementary Fig. S4 . Increased angiogenesis indices, as measured by microvessel density (MVD), were associated with a significantly worse clinical outcome ( P =0.001, log-rank test, Fig. 1f ); angiogenesis ( r =−0.268, Pearson’s two-tailed P =0.012) was inversely correlated with miR-200c expression ( Fig. 1f ). The miR-200 family regulates pro-angiogenic cytokines The miR-200 family is organized into two groups based on a single nucleotide difference in their seed sequence (group A: miR-141 and -200a; group B: miR-200b, -200c and -429), allowing each group to have overlapping and non-overlapping target genes [12] , [13] . Thus, for most of the experiments, we used a representative member from each group (miR-200a and -200b) as well as in combination, whereas for some cancer-specific experiments we chose the miR-200 member found to be most relevant based on the clinical data. We profiled 28 cancer cell lines (most from the NCI-60) for miR-200 expression levels ( Supplementary Fig. S5a ), and clones with empty vector (EV) miR-200a, miR-200b or both miR-200a and miR-200b were established for ovarian (HeyA8 and ES2) and lung (344SQ) cancer cells ( Supplementary Fig. S5b ). Global mRNA expression was analysed using a random walk-based scoring strategy [14] . An interactive angiogenesis network relevant to cancer progression emerged through regulation of IL-8 and CXCL1 ( Supplementary Fig. S6a ). IL-8 and CXCL1 are known to mediate their pro-angiogenic effects in an autocrine fashion through endothelial CXCR2 receptors [15] . Using publicly available miRNA and mRNA expression data for the NCI-60 cell line panel, we found a significant inverse correlation of miR-200c with IL-8 ( r =−0.26, Pearson’s two-tailed P =0.005; Fig. 1g ). Reverse transcriptase–PCR for a large panel of cell lines revealed a strong inverse correlation of IL-8 expression with four of the miR-200 members ( Fig. 1h , Supplementary Fig. S7 ). Importantly, based on tumour (TCGA) and cancer cell line encyclopedia data sets, the cancer types (ovarian, lung, renal and basal-like breast) in which miR-200-regulated angiogenesis were also found to have markedly elevated IL-8 and CXCL1 expression as compared with luminal breast cancers ( Fig. 2a,b , Supplementary Fig. S8a,b ). Consistent with this observation, basal-like breast cancer samples from the TCGA cohort had markedly increased IL-8 and CXCL1 expression as compared with luminal A and B subtypes ( Supplementary Fig. S8c ). As elevated levels of IL-8 have been associated with worsened clinical outcome in ovarian, renal and lung adenocarcinomas [15] , [16] , [17] , [18] , we sought to determine whether this could help explain the clinical differences seen across cancer types. Using large publicly available microarray databases [19] , in basal-like breast cancers we found that increased IL-8 expression was associated with significantly worse overall survival (hazard ratio (HR)=1.92, P =0.028, log-rank test), relapse-free survival (HR=1.48, P =0.007, log-rank test) and distant metastasis-free survival (HR=2.22, P =0.004, log-rank test), whereas these relationships were not noted in either luminal A or B subtypes ( Fig. 2c , Supplementary Fig. S8d ). Differences in clinical outcome were not observed in any breast cancer subtype based on CXCL1 expression, suggesting that miR-200 regulation of IL-8 is a key mediator explaining the divergence in clinical outcome between these breast cancer subtypes. In lung and renal cancers (notably lung adenocarcinoma), high expression of IL-8 and CXCL1 was strongly associated with worse overall survival ( Fig. 2d,e , Supplementary Fig. S8e,f ). Furthermore, on a protein level, we observed high IL-8 expression was associated with worse overall survival in ovarian cancer patients ( Fig. 2f ). 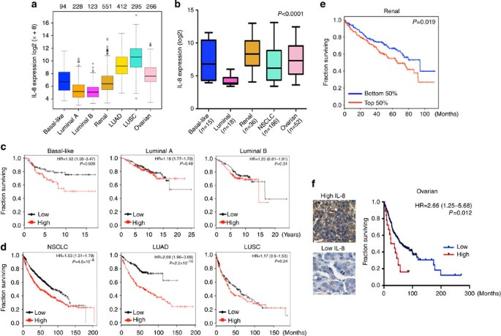Figure 2: Expression and clinical relevance of IL-8 cytokine expression. (a) Relative expression levels of IL-8 using RNA-Seq data from the TCGA data sets. The numbers above each tumour type (top of panel) represent the sample size used to calculate expression levels. LUAD, lung adenocarcinoma; LUSC, lung squamous carcinoma. Box plot represents first (lower bound) and third (upper bound) quartiles, whiskers represent 1.5 times the interquartile range. (b) Relative expression levels of IL-8 from the cancer cell line encyclopedia (CCLE) data set partitioned by designated tumour type. Analysis of variance test was used to test for statistical significance. NSCLC, non-small cell lung cancer. (c) Kaplan–Meier plots for overall survival based on IL-8 expression were generated for patients with basal-like (n=185), luminal A (n=459) and luminal B (n=308) breast cancers. (d) Kaplan–Meier plots for overall survival based on IL-8 expression for patients with NSCLC (n=1,404), lung adenocarcinoma (n=486) and LUSC (n=421). Forcandd, above (high, in red) and below (low, in black) the median expression level was used as the threshold in all cohorts. (e) Kaplan–Meier plots for overall survival based on IL-8 expression for patients with renal adenocarcinomas (n=469) from the CGA data set. Above (high, in red) and below (low, in blue) the median expression level was used as the threshold. (f) Kaplan–Meier plot for overall survival based on IL-8 protein expression for patients with ovarian cancer (n=150). Scale bars, 200 μm. Figure 2: Expression and clinical relevance of IL-8 cytokine expression. ( a ) Relative expression levels of IL-8 using RNA-Seq data from the TCGA data sets. The numbers above each tumour type (top of panel) represent the sample size used to calculate expression levels. LUAD, lung adenocarcinoma; LUSC, lung squamous carcinoma. Box plot represents first (lower bound) and third (upper bound) quartiles, whiskers represent 1.5 times the interquartile range. ( b ) Relative expression levels of IL-8 from the cancer cell line encyclopedia (CCLE) data set partitioned by designated tumour type. Analysis of variance test was used to test for statistical significance. NSCLC, non-small cell lung cancer. ( c ) Kaplan–Meier plots for overall survival based on IL-8 expression were generated for patients with basal-like ( n =185), luminal A ( n =459) and luminal B ( n =308) breast cancers. ( d ) Kaplan–Meier plots for overall survival based on IL-8 expression for patients with NSCLC ( n =1,404), lung adenocarcinoma ( n =486) and LUSC ( n =421). For c and d , above (high, in red) and below (low, in black) the median expression level was used as the threshold in all cohorts. ( e ) Kaplan–Meier plots for overall survival based on IL-8 expression for patients with renal adenocarcinomas ( n =469) from the CGA data set. Above (high, in red) and below (low, in blue) the median expression level was used as the threshold. ( f ) Kaplan–Meier plot for overall survival based on IL-8 protein expression for patients with ovarian cancer ( n =150). Scale bars, 200 μm. Full size image Next, we examined whether IL-8 and CXCL1 are direct targets of the miR-200 family. In ES2 and HeyA8 cells, we found IL-8 and CXCL1 levels were reduced by miR-200a and -200b-expressing clones ( Fig. 3a ). As mice only produce CXCL1 (an IL-8 homologue), we found miR-200 regulation of CXCL1 appears to be conserved across species ( Fig. 3b , Supplementary Fig. S6b ). Following transfection of several ovarian, lung, renal and breast (luminal and basal-like) cell lines with various miR-200 members, we found variable degrees of knockdown of IL-8 ( Supplementary Fig. S9a ). In addition, in two high miR-200-expressing cell lines, treatment with miR-200b and -200c inhibitors led to increased expression of IL-8 and CXCL1 ( Supplementary Fig. S9b ). We also investigated whether miR-200 can directly affect angiogenesis by targeting endothelial cell production of IL-8 and CXCL1 . There were significant reductions in the expression of both pro-angiogenic factors after transfection with either miR-200a or -200b in RF24 endothelial cells, especially in comparison with a previously identified endothelial miR-200b target, Ets-1 (ref. 20 ; Fig. 3c ). Enzyme-linked immunosorbent assay (ELISA) of supernatants after 48 h of transient transfection for each cell line ( Fig. 3d,e ) and for stable HeyA8 clones ( Fig. 3f ) confirmed reductions in IL-8 and CXCL1 protein levels. Vascular endothelial growth factor-A ( VEGFa ), a previously reported miR-200b target [21] , was reduced at a transcript level in ES2 (not HeyA8), but was not decreased by ELISA assay ( Supplementary Fig. S10 ). 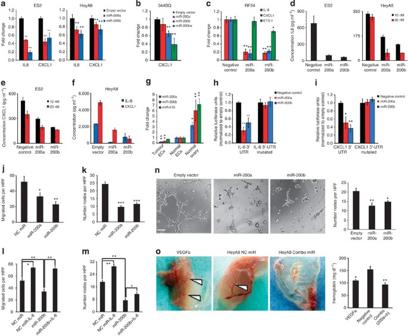Figure 3: Direct and indirect anti-angiogenic effects by miR-200. (a) Expression levels of IL-8 and CXCL1 for ES2 and HeyA8 clones,n=3. Data are averages±s.e.m. (b) Expression levels of CXCL1 from murine lung cancer (344SQ) clones,n=3. Data are averages±s.e.m. (c) Expression levels of IL-8, CXCL1 and Ets-1 following transfection of RF24 cells. Data are averages±s.e.m.,n=3. (d) ELISA for IL-8 (ES2 and HeyA8) and (e) CXCL1 (ES2) following transfection. Data are averages±s.e.m.,n=3. (f) ELISA for IL-8 and CXCL1 supernatants from HeyA8 clones. Data are averages±s.e.m.,n=3. (g) Relative expression levels of miR-200a, miR-200b and miR-210 in clinically isolated endothelial cells from normal ovary (n=2) versus carcinoma (n=6). Further comparison with normal ovarian epithelium (n=2) is shown. Data are averages±s.e.m.P-values obtained with Mann–Whitney’st-test. (h) Relative luciferase activity normalized to empty control for the IL-8 3′-untranslated region (UTR) (wild-type, left; mutated, right). Data are averages±s.e.m.P-values obtained with Student’st-test,n=6. (i) Relative luciferase activity normalized to empty control for the CXCL1 3′-UTR (wild-type, left; mutated, right). Data are averages±s.e.m.P-values obtained with Student’st-test,n=6. (j) Direct effects on migration,n=4 and (k) tube formation,n=6 following RF24 transfection. Data are averages±s.e.m.P-values were with Student’st-test. (l) Effects of exogenous recombinant IL-8 (10 ng ml−1) on migration and (m) tube formation following RF24 transfection,n=6. Data are averages±s.e.m.P-values were with Student’st-test. (n) Indirect effects on RF24 tube formation following incubation with HeyA8 supernatants,n=6. Data are averages±s.e.m.P-values were obtained with Student’st-test. Scale bar, 500 μm. (o) Representative images (left) and haemoglobin quantification (right) of anin-vivomatrigel plug assay,n=2. White arrows demonstrate new blood vessel formation. Data are averages±s.e.m.P-values obtained with Student’st-test. *P<0.05, **P<0.01, ***P<1 × 10−9. Figure 3: Direct and indirect anti-angiogenic effects by miR-200. ( a ) Expression levels of IL-8 and CXCL1 for ES2 and HeyA8 clones, n =3. Data are averages±s.e.m. ( b ) Expression levels of CXCL1 from murine lung cancer (344SQ) clones, n =3. Data are averages±s.e.m. ( c ) Expression levels of IL-8, CXCL1 and Ets-1 following transfection of RF24 cells. Data are averages±s.e.m., n =3. ( d ) ELISA for IL-8 (ES2 and HeyA8) and ( e ) CXCL1 (ES2) following transfection. Data are averages±s.e.m., n =3. ( f ) ELISA for IL-8 and CXCL1 supernatants from HeyA8 clones. Data are averages±s.e.m., n =3. ( g ) Relative expression levels of miR-200a, miR-200b and miR-210 in clinically isolated endothelial cells from normal ovary ( n =2) versus carcinoma ( n =6). Further comparison with normal ovarian epithelium ( n =2) is shown. Data are averages±s.e.m. P -values obtained with Mann–Whitney’s t -test. ( h ) Relative luciferase activity normalized to empty control for the IL-8 3′-untranslated region (UTR) (wild-type, left; mutated, right). Data are averages±s.e.m. P -values obtained with Student’s t -test, n =6. ( i ) Relative luciferase activity normalized to empty control for the CXCL1 3′-UTR (wild-type, left; mutated, right). Data are averages±s.e.m. P -values obtained with Student’s t -test, n =6. ( j ) Direct effects on migration, n =4 and ( k ) tube formation, n =6 following RF24 transfection. Data are averages±s.e.m. P -values were with Student’s t -test. ( l ) Effects of exogenous recombinant IL-8 (10 ng ml −1 ) on migration and ( m ) tube formation following RF24 transfection, n =6. Data are averages±s.e.m. P -values were with Student’s t -test. ( n ) Indirect effects on RF24 tube formation following incubation with HeyA8 supernatants, n =6. Data are averages±s.e.m. P -values were obtained with Student’s t -test. Scale bar, 500 μm. ( o ) Representative images (left) and haemoglobin quantification (right) of an in-vivo matrigel plug assay, n =2. White arrows demonstrate new blood vessel formation. Data are averages±s.e.m. P -values obtained with Student’s t -test. * P <0.05, ** P <0.01, *** P <1 × 10 −9 . Full size image Next, we compared the relative miR-200 expression levels of both murine and human endothelial cells (MOEC and RF24, respectively) with EMT-positive (344SQ, ES2 and HeyA8) and epithelial (SKOV3ip1) miR-200-expressing carcinoma cell lines [2] , [22] ; both endothelial cell lines had very low miR-200a and miR-200b expression ( Supplementary Fig. S11 ). In contrast with miR-210, which is known to regulate angiogenesis under hypoxia [23] , endothelial cells isolated directly from human ovarian cancers had significantly lower miR-200 expression than normal endothelial cells ( Fig. 3g ), suggesting a potential direct role for miR-200 in cancer-related angiogenesis. To validate that IL-8 and CXCL1 are direct miR-200 targets, luciferase assays using the entire 3′-untranslated region were performed. As compared with cells transfected with negative control miRNA, the relative luciferase activity for IL-8 and CXCL1 were significantly reduced by both miR-200a and miR-200b ( Fig. 3h,i ). The putative binding sites for miR-200a and miR-200b were predicted for IL-8 and CXCL1 , using several bioinformatic algorithms ( Supplementary Fig. S12 ). For both genes, mutation of the binding site at the seed sequence for miR-200a and miR-200b abrogated knockdown, indicating these are direct miR-200 targets ( Fig. 3h,i ). Following miR-200 transfection, RF24 cells had significantly decreased migration ( Fig. 3j ) and tube formation capability ( Fig. 3k ), which was not due to altered cell viability ( Supplementary Fig. S13 ). Transfection with miR-200a or -200b resulted in endothelial cells with blunting of pseudopodia and a more rounded shape than those in controls ( Supplementary Fig. S14 ). Although exogenous recombinant IL-8 was able to rescue the miR-200b effects on migration ( Fig. 3l ), only a partial rescue was observed for tube formation ( Fig. 3m ), suggesting other target genes are involved in this process. In addition, to assess for indirect effects of secreted IL-8 and CXCL1 on angiogenesis, we used conditioned media from HeyA8 clones ( Fig. 3f ) and found that tube formation was significantly decreased with supernatants from both miR-200a- and -200b-expressing cells ( Fig. 3n ). Next, using an in-vivo matrigel plug assay, we compared the indirect effects of miR-200 on angiogenesis using conditioned media from HeyA8 cell lines ( Supplementary Fig. S15 ). Compared with VEGFa (positive control) and negative control miRNA-treated cells, the combination of miR-200a and -200b led to substantial reductions in MVD ( Fig. 3o ) and haemoglobin content ( P =5 × 10 −4 , Student’s t -test), a surrogate for functional blood flow ( Fig. 3o ). miR-200 members regulate tumour angiogenesis We then examined the biological effects of in-vivo miRNA delivery using well-characterized nanoparticle platforms [24] , [25] . With the neutral 1,2-dioleoyl-sn-glycero-3-phosphatidylcholine (DOPC) nanoliposomes [24] , a single dose of miR-200b by tail vein injection decreased a well-validated target, ZEB1 , and increased E-cadherin expression in a subcutaneous lung cancer model (344SQ; Fig. 4a–d ). Using Quasar 570-labelled oligonucleotides injected intravenously (i.v.) into mice bearing subcutaneous 344SQ tumours, we found delivery within the tumour and beyond the vasculature ( Fig. 4e ). 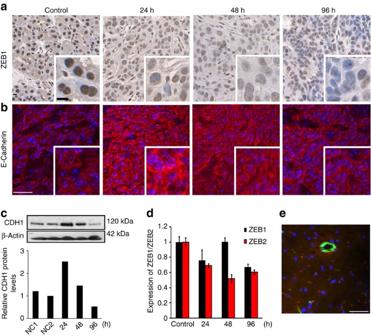Figure 4: Effective target modulation with systemic miR-200 delivery. (a) Compared with an untreated 344SQ tumour, ZEB1 immunohistochemistry and (b) E-Cadherin immunofluorescent staining intensities following systemic miR-200b delivery. (c) Immunoblotting of tumour lystates for E-Cadherin (CDH1). (d) Relative tumour ZEB1 and ZEB2 expression levels following delivery. Data are averages±s.e.m.,n=3. (e) Deep tumour delivery of Quasar 570-labelled (red) control miRNA in DOPC beyond the vasculature (CD31 staining—green, nuclear staining with Hoechst 33342—blue). Similar to a prior report24, ~80% of the fields had nanoparticle delivery, and within each field 35% of tumour cells contained signal. Scale bars, 100 μm (a+e); 50 μm (b). Figure 4: Effective target modulation with systemic miR-200 delivery. ( a ) Compared with an untreated 344SQ tumour, ZEB1 immunohistochemistry and ( b ) E-Cadherin immunofluorescent staining intensities following systemic miR-200b delivery. ( c ) Immunoblotting of tumour lystates for E-Cadherin (CDH1). ( d ) Relative tumour ZEB1 and ZEB2 expression levels following delivery. Data are averages±s.e.m., n =3. ( e ) Deep tumour delivery of Quasar 570-labelled (red) control miRNA in DOPC beyond the vasculature (CD31 staining—green, nuclear staining with Hoechst 33342—blue). Similar to a prior report [24] , ~80% of the fields had nanoparticle delivery, and within each field 35% of tumour cells contained signal. Scale bars, 100 μm ( a + e ); 50 μm ( b ). Full size image Next, to assess miR-200 effects on tumour growth, EV and miR-200-transfected lung cancer cells (344SQ) were injected subcutaneously (s.c.; ten mice per group). As compared with EV, clones expressing miR-200a or -200b led to decreased tumour volume by 55% and 51%, respectively, whereas clones expressing miR-200ba led to a 69% reduction ( P =0.027, Student’s t -test, Fig. 5a ). We determined the effects of systemic delivery of miR-200 members incorporated in DOPC nanoliposomes; 1 week after s.c. injection of 344SQ cells, mice were randomly assigned to the following groups: (1) control miRNA-DOPC, (2) miR-200a-DOPC, (3) miR-200b-DOPC and (4) miR-200a+miR-200b-DOPC. Following 2 weeks of treatment, although miR-200a and -200b led to reductions in tumour volumes of 25% and 36%, respectively, the combination led to a reduction in volume of 72% ( P =0.002, Student’s t -test, Fig. 5b ). For both in-vivo experiments, reduced tumour volumes corresponded with significant reductions in tumour mass ( Supplementary Fig. S16 ). Significant reduction in MVD was noted in the models with stably-expressing ( Fig. 5c ) and DOPC-delivered miR-200 family members ( Fig. 5c ). In addition, delivery of miR-200 family members also led to reductions in proliferation ( Fig. 5d ). Additional in-vivo experiments were carried out in ovarian (HeyA8) and renal (A498) cancer models using miR-200 members found to have prognostic significance ( Fig. 1a ). Following 2 weeks of treatment, compared with control miRNA, miR-200c-DOPC led to a 60% reduction in tumour mass ( P =0.03, Student’s t -test, Fig. 5e ). Similarly, for the renal cancer model, systemic delivery of miR-200a and -200b led to a 90% reduction in tumour mass ( P =0.019, Student’s t -test, Fig. 5f ). 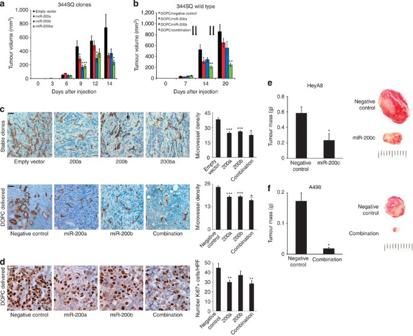Figure 5: Effects of miR-200 delivery on angiogenesis in several cancer types. (a) Tumour volumes in a lung cancer model of 344SQ clones,n=10 per group (no treatment), and (b) 344SQ wild-type cells (treated with systemic miRNAs incorporated into DOPC),n=10 per group. Data are averages±s.e.m.P-values obtained with Student’st-test. (c) CD31 staining and microvessel density scoring for (top) stable clones or (bottom) wild-type 344SQ tumours following miRNA delivery. Bar graphs represent number of microvessels per high-powered field (hpf),n=5 tumours per group. Scale bars, 500 μm. Data are averages±s.e.m.P-values obtained with Student’st-test. (d) Ki-67 staining for 344SQ tumours following miRNA delivery. Bar graphs represent number of Ki-67 staining cells per hpf,n=5 tumours per group. Scale bar, 200 μm. Data are averages±s.e.m.P-values obtained with Student’st-test. (e) Mass of HeyA8 ovarian tumours following treatment with either control miRNA or miR-200c, and (f) mass of A498 renal tumours following treatment with control miRNA or both miR-200a and miR-200b,n=5 per group for each experiment. Data are averages±s.e.m. Representative tumours are shown, scale in mm. *P<0.05, **P<0.01, ***P<1 × 10−5, ±P<1 × 10−8. Figure 5: Effects of miR-200 delivery on angiogenesis in several cancer types. ( a ) Tumour volumes in a lung cancer model of 344SQ clones, n =10 per group (no treatment), and ( b ) 344SQ wild-type cells (treated with systemic miRNAs incorporated into DOPC), n =10 per group. Data are averages±s.e.m. P -values obtained with Student’s t -test. ( c ) CD31 staining and microvessel density scoring for (top) stable clones or (bottom) wild-type 344SQ tumours following miRNA delivery. Bar graphs represent number of microvessels per high-powered field (hpf), n =5 tumours per group. Scale bars, 500 μm. Data are averages±s.e.m. P -values obtained with Student’s t -test. ( d ) Ki-67 staining for 344SQ tumours following miRNA delivery. Bar graphs represent number of Ki-67 staining cells per hpf, n =5 tumours per group. Scale bar, 200 μm. Data are averages±s.e.m. P -values obtained with Student’s t -test. ( e ) Mass of HeyA8 ovarian tumours following treatment with either control miRNA or miR-200c, and ( f ) mass of A498 renal tumours following treatment with control miRNA or both miR-200a and miR-200b, n =5 per group for each experiment. Data are averages±s.e.m. Representative tumours are shown, scale in mm. * P <0.05, ** P <0.01, *** P <1 × 10 −5 , ± P <1 × 10 −8 . Full size image Therapeutic effects of miR-200 in metastatic models To determine whether DOPC can effectively deliver miRNA to an orthotopic lung cancer model (344SQ), as well as to distant metastases, we utilized fluorescence imaging. Using Cy5.5-labelled oligonucleotides DOPC [25] , both i.v. and intraperitoneal (i.p.) routes were effective in delivering oligonucleotides into all sites of disease ( Fig. 6a,b ), including metastatic lesions in the spleen and liver [26] ( Fig. 6c,d ). To determine the therapeutic efficacy of miR-200 delivery, we used orthotopic models (lung, ovarian and basal-like breast) that readily form metastasis. For the lung cancer model (344SQ), delivery of miR-200a and -200b members resulted in a significant decrease in primary tumour burden as compared with control miRNA ( Fig. 7a ). In addition, significant reductions in the number and aggregate mass of distant metastases were observed in all groups ( Fig. 7b ). Although the tumours metastasized to common sites for lung cancer in the control miRNA group ( Fig. 7c ), significant reductions in common metastatic regions were observed for all treatment groups ( Fig. 7d ). 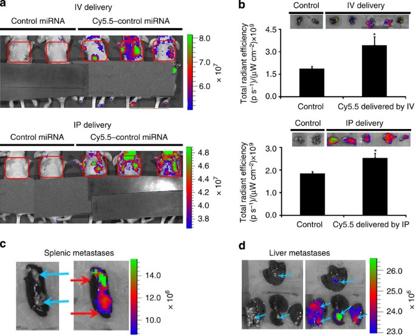Figure 6: Nanoparticle delivery of oligonucleotides in a metastatic lung cancer model. Two weeks following injection with the 344SQ cell line, mice were treated with either DOPC/Cy5.5-labelled or DOPC/non-labelled oligonucleotides (200 μg kg−1per mouse, 6 mice per group) by either intravenous (i.v.) or intraperitoneal (i.p.) routes. (a) Forty-eight hours after treatment, mice in each group were imaged adjacently before killing. Cy5.5-lablelled groups demonstrated enhanced uptake by either delivery route. (b) Excised primary lung tumours demonstrated increased uptake by measurement of total radiant efficiency (p s−1)/(μW cm−2). Gross metastatic lesions in the (c) spleen and in several (d) liver lesions demonstrated notable Cy5.5 uptake, suggesting DOPC-delivered oligonucleotides can target metastasis. Data are averages±s.e.m.,n=6,P-values obtained with Student’st-test. *P<0.001. Figure 6: Nanoparticle delivery of oligonucleotides in a metastatic lung cancer model. Two weeks following injection with the 344SQ cell line, mice were treated with either DOPC/Cy5.5-labelled or DOPC/non-labelled oligonucleotides (200 μg kg −1 per mouse, 6 mice per group) by either intravenous (i.v.) or intraperitoneal (i.p.) routes. ( a ) Forty-eight hours after treatment, mice in each group were imaged adjacently before killing. Cy5.5-lablelled groups demonstrated enhanced uptake by either delivery route. ( b ) Excised primary lung tumours demonstrated increased uptake by measurement of total radiant efficiency (p s −1 )/(μW cm − 2 ). Gross metastatic lesions in the ( c ) spleen and in several ( d ) liver lesions demonstrated notable Cy5.5 uptake, suggesting DOPC-delivered oligonucleotides can target metastasis. Data are averages±s.e.m., n =6, P -values obtained with Student’s t -test. * P <0.001. 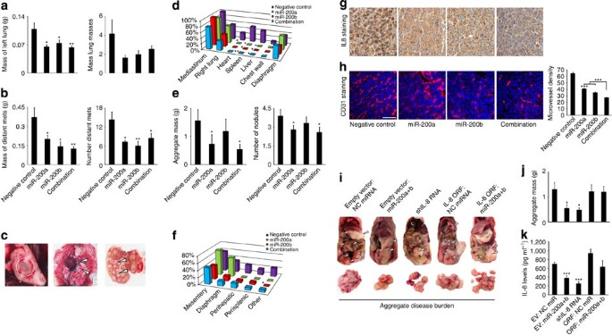Figure 7: Therapeutic effects of miR-200 delivery in metastatic models. (a) Average mass of the left lung (left) and number of lung nodules (right) in the 344SQ lung cancer model. Data are averages±s.e.m.,n=10.P-values obtained with Student’st-test. (b) Average aggregate mass of distant metastases (left) and number of distant metastases (right),n=10 per group. Data are averages±s.e.m.P-values were obtained with Student’st-test. (c) Representative images of an orthotopic left lung tumour (left, encircled), mediastinal (middle, arrows) and liver metastases (right, arrows). (d) Frequency of lung cancer metastases.P-values obtained withχ2-test. (e) Aggregate mass of distant metastases (left) and number of metastases (right) in the HeyA8 ovarian cancer model,n=10 per group, Data are averages±s.e.m. (f) Frequency of metastases to distant sites. Other: the pelvis, ovary, kidney or liver. (g) Representative tumour staining of IL-8 in the HeyA8 model. Scale bar, 200 μm. (h) Microvessel density for HeyA8 tumours following miRNA delivery,n=5 tumours per group. Data are averages±s.e.m.P-values obtained with Student’st-test. Scale bar, 200 μm. (i) Representative images of grossin vivo(top, white arrows) and aggregateex vivo(bottom) metastatic tumour burden in the HeyA8 ovarian model at the time of necropsy. (j) Aggregate mass of metastasis (n=10 mice per group) and (k) IL-8 plasma levels (n=5 per group) in the HeyA8 model. Data are averages±s.e.m.P-values obtained with Student’st-test. *P<0.05, **P<0.01, ***P<1 × 10−4, ±P<1 × 10−6. Full size image Figure 7: Therapeutic effects of miR-200 delivery in metastatic models. ( a ) Average mass of the left lung (left) and number of lung nodules (right) in the 344SQ lung cancer model. Data are averages±s.e.m., n =10. P -values obtained with Student’s t -test. ( b ) Average aggregate mass of distant metastases (left) and number of distant metastases (right), n =10 per group. Data are averages±s.e.m. P -values were obtained with Student’s t -test. ( c ) Representative images of an orthotopic left lung tumour (left, encircled), mediastinal (middle, arrows) and liver metastases (right, arrows). ( d ) Frequency of lung cancer metastases. P -values obtained with χ 2 -test. ( e ) Aggregate mass of distant metastases (left) and number of metastases (right) in the HeyA8 ovarian cancer model, n =10 per group, Data are averages±s.e.m. ( f ) Frequency of metastases to distant sites. Other: the pelvis, ovary, kidney or liver. ( g ) Representative tumour staining of IL-8 in the HeyA8 model. Scale bar, 200 μm. ( h ) Microvessel density for HeyA8 tumours following miRNA delivery, n =5 tumours per group. Data are averages±s.e.m. P -values obtained with Student’s t -test. Scale bar, 200 μm. ( i ) Representative images of gross in vivo (top, white arrows) and aggregate ex vivo (bottom) metastatic tumour burden in the HeyA8 ovarian model at the time of necropsy. ( j ) Aggregate mass of metastasis ( n =10 mice per group) and ( k ) IL-8 plasma levels ( n =5 per group) in the HeyA8 model. Data are averages±s.e.m. P -values obtained with Student’s t -test. * P <0.05, ** P <0.01, *** P <1 × 10 −4 , ± P <1 × 10 −6 . Full size image Similarly, for the ovarian cancer model (HeyA8), the delivery of miR-200 members resulted in a significant decrease in total metastatic burden as compared with control miRNA ( Fig. 7e ). Metastatic lesions were decreased in common metastatic sites of high-grade serous ovarian carcinoma ( Fig. 7f ). By profiling tumours from the control miRNA and combination groups for miR-200a, we observed that the increase of miR-200a (18-fold increase) in the combination group was comparable with that observed in ovarian cancer cell lines with relatively normal (SKOV3ip1, 9-fold increase over HeyA8) and elevated (A2774, 38-fold increase over HeyA8) miR-200a levels ( Supplementary Fig. S17 ). This suggests that a therapeutic benefit may be realized by increasing a tumour’s miR-200 expression to levels more comparable with epithelial cancer cell lines ( Supplementary Fig. S5a ). Reduced tumour expression of IL-8 was observed in all treatment groups ( Fig. 7g ). This corresponded with significant reductions in angiogenesis, most notably in the combination group ( Fig. 7h ). We observed no significant associations with miR-200 treatment and pericyte coverage of blood vessels ( Supplementary Fig. S18 ). To establish whether there is a causal link between miR-200 targeting of IL-8 and the observed therapeutic effects, we developed the following HeyA8 ovarian clones: -EV, IL-8 shRNA and IL-8 open-reading frame (ORF). Five days following i.p. injection of cancer cells, mice were assigned to the following groups ( n =10 per group)—(1) EV: control miRNA-DOPC; (2) EV: miR-200a+miR-200b-DOPC; (3) shIL-8; (4) IL-8 ORF: control miRNA-DOPC; and (5) IL-8 ORF: miR-200a+miR-200b-DOPC. After 3 weeks of treatment, a necropsy was performed. Importantly, as compared with the EV: control miRNA group, aggregate disease burden was significantly reduced in the EV: miR-200a+miR-200b-DOPC (57%, P =0.045, Student’s t -test) and shIL-8 (63%, P =0.012, Student’s t -test) groups ( Fig. 7j ). Conversely, miR-200a+miR-200b-DOPC delivery in the IL-8 ORF groups did not lead to any reduction in disease burden ( Fig. 7j ). Consistent with these findings, IL-8 plasma levels were only significantly reduced in the EV: miR-200a+miR-200b-DOPC (46%, P <0.0001, Student’s t -test) and shIL-8 (63%, P <0.0001, Student’s t -test) groups ( Fig. 7k ). In addition, circulating IL-8 plasma levels strongly correlated with aggregate disease burden ( r =0.77, Spearman’s two-sided P <0.0001, Supplementary Fig. S19 ). Together, these data strongly implicate IL-8 targeting to account for miR-200’s therapeutic effects. Furthermore, plasma IL-8 levels may serve as a novel candidate biomarker for miR-200-based delivery. Consistent with our TCGA and cancer cell line encyclopedia analysis, compared with luminal breast cancer, basal-like cell lines were found to have substantially lower miR-200 and markedly increased IL-8 and CXCL1 expression levels ( Fig. 8a ). On the basis of our clinical findings ( Supplementary Fig. S1b ) and a prior report showing miR-200 members can promote hormone-positive breast cancers [4] , we assessed whether miR-141 could instead result in therapeutic effects in a basal-like breast cancer model. One week following orthotopic injection of BT-549 cells, mice were randomly assigned to the following groups ( n =10 per group): (1) control miRNA-DOPC or (2) miR-141-DOPC. Following 2 weeks of treatment, compared with controls, miR-141 treatment led to a 49% reduction in primary tumour growth ( P =0.05, Student’s t -test, Fig. 8b ), and resected primary tumours exhibited a 22% reduction in MVD ( P <0.0001, Student’s t -test). This was associated with significant reductions in the primary tumour expression of IL-8 and CXCL1 ( Fig. 8c ). Two weeks following primary tumour removal, miR-141 led to significant reductions in the frequency of gross peritoneal ( P =0.03, χ 2 -test) and microscopic lung ( P =0.008, χ 2 -test) metastases ( Fig. 8d ). 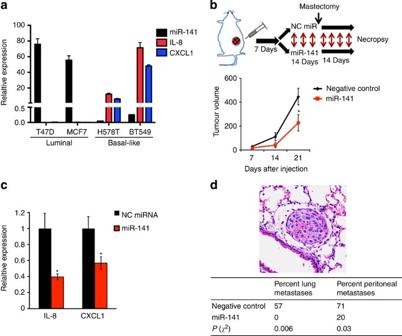Figure 8: Therapeutic effects of miR-200 in a basal-like breast cancer model. (a) Relative expression levels of miR-141, IL-8 and CXCL1 in breast cell lines. Data are averages±s.e.m.,n=3. (b) Schematic of basal-like experiment (top) and primary tumour volumes (bottom) following systemic miRNA delivery. Data are averages±s.e.m.,n=10.P-values obtained with Student’st-test. (c) Relative expression level of IL-8 and CXCL1 in resected primary tumours (n=4) from each treatment group. (d) Haematoxylin and eosin image of lung micrometastasis (top) and frequencies of peritoneal and microscopic lung metastases (bottom).P-values obtained with theχ2-test. *P<0.05. Figure 8: Therapeutic effects of miR-200 in a basal-like breast cancer model. ( a ) Relative expression levels of miR-141, IL-8 and CXCL1 in breast cell lines. Data are averages±s.e.m., n =3. ( b ) Schematic of basal-like experiment (top) and primary tumour volumes (bottom) following systemic miRNA delivery. Data are averages±s.e.m., n =10. P -values obtained with Student’s t -test. ( c ) Relative expression level of IL-8 and CXCL1 in resected primary tumours ( n =4) from each treatment group. ( d ) Haematoxylin and eosin image of lung micrometastasis (top) and frequencies of peritoneal and microscopic lung metastases (bottom). P -values obtained with the χ 2 -test. * P <0.05. Full size image Direct anti-angiogenesis effects Because of the in-vitro effects of miR-200 on endothelial function, we used chitosan nanoparticles to directly deliver miRNA to the tumour vasculature ( Fig. 9a ). To assess the direct (tumour endothelium) and indirect (tumour secretion of IL-8 and CXCL1) effects of miR-200 on angiogenesis, we used the metastatic HeyA8 model. Notably, delivery of miR-200a and -200b resulted in a 92% reduction in metastatic burden as compared with control miRNA ( P =0.002, Student’s t -test, Fig. 9b ). To further assess the vascular effects of direct and indirect targeting, 2 weeks after injecting mice with HeyA8 ovarian cell lines, we delivered three serial doses of chitosan nanoparticles containing either control miRNA or the combination of miR-200a and -200b. Tumour vasculature following miR-200 treatment was significantly less permeable ( Fig. 9c ), and the vessels were more organized and less tortuous than the control miRNA group ( Fig. 9d ). 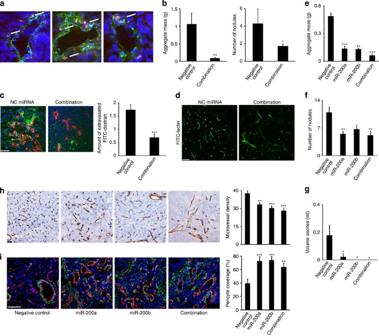Figure 9: Direct angiogenesis targeting and vascular normalization by endothelial miR-200 delivery. (a) Intra-endothelial and peri-endothelial miRNA localization (arrows) in HeyA8 tumours. Vessels visualized with CD31 (green) staining, Cy3-miRNA signal (red) and nuclei visualized with Hoechst 33342 (blue). Scale bar, 100 μm. (b) Average aggregate mass of distant metastases (left) and number of metastases (right) in HeyA8 ovarian model,n=10 per group. Data are averages±s.e.m.P-values obtained with Student’st-test. (c) Representative images (left) of FITC-dextran (green), CD31 (red) and nuclei visualized with Hoechst 33342 (blue) in HeyA8 tumours following three serial deliverys of miRNAs (n=3 mice per group). Scale bar, 100 μm. Bar graphs (right) show a quantitative analysis of extravascular FITC-dextran. Data are averages±s.e.m. (d) Representative confocal images of tumour vessels labelled with FITC-lectin in HeyA8 tumours following three serial deliverys of miRNAs (n=2 mice per group). Scale bar, 50 μm. (e) Average aggregate mass of distant metastases and (f) number of metastases for the A2774 ovarian cancer model,n=10 per group. Data are averages±s.e.m.P-values obtained with Student’st-test. (g) Average volume of peritoneal ascites in the A2774 model, measured in ml. (h) Representative CD31 staining and microvessel density scoring for A2774 tumours following miRNA delivery. Bar graphs represent number of microvessels per hpf,n=5 tumours per group. Scale bar, 500 μm. (i) Images of dual desmin and CD31 staining and percentage of pericyte coverage for A2774 tumours following miRNA delivery. Bar graphs represent the percentage of pericyte-covered microvessels per hpf,n=5 tumours per group. Scale bar, 100 μm. Data are averages±s.e.m. *P≤0.05, **P<0.01, ***P<0.001. Figure 9: Direct angiogenesis targeting and vascular normalization by endothelial miR-200 delivery. ( a ) Intra-endothelial and peri-endothelial miRNA localization (arrows) in HeyA8 tumours. Vessels visualized with CD31 (green) staining, Cy3-miRNA signal (red) and nuclei visualized with Hoechst 33342 (blue). Scale bar, 100 μm. ( b ) Average aggregate mass of distant metastases (left) and number of metastases (right) in HeyA8 ovarian model, n =10 per group. Data are averages±s.e.m. P -values obtained with Student’s t -test. ( c ) Representative images (left) of FITC-dextran (green), CD31 (red) and nuclei visualized with Hoechst 33342 (blue) in HeyA8 tumours following three serial deliverys of miRNAs ( n =3 mice per group). Scale bar, 100 μm. Bar graphs (right) show a quantitative analysis of extravascular FITC-dextran. Data are averages±s.e.m. ( d ) Representative confocal images of tumour vessels labelled with FITC-lectin in HeyA8 tumours following three serial deliverys of miRNAs ( n =2 mice per group). Scale bar, 50 μm. ( e ) Average aggregate mass of distant metastases and ( f ) number of metastases for the A2774 ovarian cancer model, n =10 per group. Data are averages±s.e.m. P -values obtained with Student’s t -test. ( g ) Average volume of peritoneal ascites in the A2774 model, measured in ml. ( h ) Representative CD31 staining and microvessel density scoring for A2774 tumours following miRNA delivery. Bar graphs represent number of microvessels per hpf, n =5 tumours per group. Scale bar, 500 μm. ( i ) Images of dual desmin and CD31 staining and percentage of pericyte coverage for A2774 tumours following miRNA delivery. Bar graphs represent the percentage of pericyte-covered microvessels per hpf, n =5 tumours per group. Scale bar, 100 μm. Data are averages±s.e.m. * P ≤0.05, ** P <0.01, *** P <0.001. Full size image To assess potential therapeutic effects of direct endothelial targeting, we chose the A2774 model because of high baseline miR-200 levels. Furthermore, although miR-200 transfection in A2774 cells led to modest reductions in IL-8 and CXCL1 , these reductions would be considered inconsequential given their baseline expression being markedly lower than ES2 and HeyA8 ( Supplementary Fig. S20 ). To further enhance tumour endothelial targeting, we used RGD-labelled chitosan nanoparticles, which bind to αvβ3 integrin [27] . Compared with control miRNA, the delivery of miR-200 members resulted in a marked decrease in tumour burden (all P <0.01, Student’s t -test, Fig. 9e ). This also corresponded with decreases in the total number of metastases ( Fig. 9f ) and ascites compared with control miRNA ( Fig. 9g ). There was no apparent toxicity observed in mice from any treatment group based on feeding habits, body weight or activity. MiR-200 delivery led to significant reductions in MVD as compared with control miRNA ( Fig. 9h ). Compared with control miRNA, we observed a near doubling in pericyte coverage in tumours from all miR-200 treatment groups ( P <0.01 for all miR-200 groups, Student’s t -test, Fig. 9i ), suggesting a role of miR-200 in blood vessel maturation. Consistent with these findings, increased pericyte coverage has been related to metastasis inhibition [28] . Although the mechanism of vascular normalization is likely multifactorial [29] , including decreased IL-8 and CXCL1 , we also observed increased migration of 10T1/2 pericyte-like cells using conditioned media from miR-200-transfected cells ( Fig. 10a,b ), which was unrelated to IL-8 levels ( Fig. 10c ). Taken together, we have demonstrated miR-200’s role in targeting angiogenesis through direct and indirect mechanisms ( Fig. 10d ) in a cancer-type-dependent context. 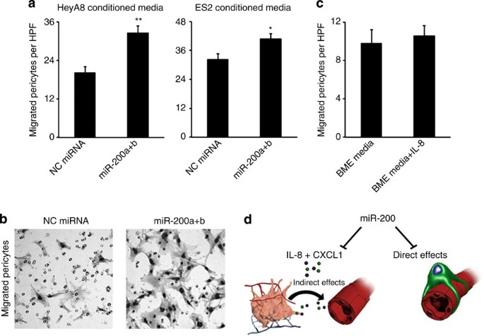Figure 10: Migration of pericyte-like cells using conditioned media of miR-200-transfected cells. (a) Migration of 10T1/2 pericyte-like cells at 6 h using conditioned media from HeyA8 (left) and ES2 (right) cells following miRNA transfection as a chemo-attractant. Data are averages±s.e.m.,n=2.P-values obtained with Student’st-test. (b) Migration of 10T1/2 cells using complete media or complete media plus 10 ng ml−1of IL-8 as a chemo-attractant. Data are averages±s.e.m.,n=2.P-values obtained with Student’st-test. (c) Representative images of migrated pericyte-like cells using conditioned media from HeyA8 cells. (d) A model for miR-200 targeting of direct and indirect effects on angiogenesis. *P<0.05, **P<0.001. Figure 10: Migration of pericyte-like cells using conditioned media of miR-200-transfected cells. ( a ) Migration of 10T1/2 pericyte-like cells at 6 h using conditioned media from HeyA8 (left) and ES2 (right) cells following miRNA transfection as a chemo-attractant. Data are averages±s.e.m., n =2. P -values obtained with Student’s t -test. ( b ) Migration of 10T1/2 cells using complete media or complete media plus 10 ng ml −1 of IL-8 as a chemo-attractant. Data are averages±s.e.m., n =2. P -values obtained with Student’s t -test. ( c ) Representative images of migrated pericyte-like cells using conditioned media from HeyA8 cells. ( d ) A model for miR-200 targeting of direct and indirect effects on angiogenesis. * P <0.05, ** P <0.001. Full size image In addition to regulating EMT, the miR-200 family functions as a master regulator of several cancer hallmarks [30] , [31] . Several reports have linked low miR-200 levels with increased chemotherapy and anti-epidermal growth factor receptor therapy resistance and increased expression of TUBB3 (ref. 32 ), SUZ12 (ref. 30 ), ERRFI-1 (ref. 33 ) and ZEB1/2 (ref. 34 ). By targeting FAP-1 , miR-200 has been found to induce apoptosis through upregulating CD95 (ref. 35 ). These studies suggest that miR-200 has important roles in cancer progression and may have therapeutic potential. However, miR-200 overexpression in a breast cancer model promoted distant metastasis [5] , suggesting possible differences based on cancer subtype. Through a systematic analysis of clinical data sets, we unexpectedly found profound differences in overall survival between common cancer types based on the expression of miR-200 family members. Similar to prior reports in hormone-positive breast cancers [4] , we found high miR-200 members associated with worse outcome in luminal breast cancers. Uniquely, however, extensive data analyses revealed strong miR-200 regulation of angiogenesis networks in ovarian, lung, renal and basal-like breast adenocarcinomas. Subsequent in-vitro and in-vivo experiments validated miR-200’s role in regulating angiogenesis by directly targeting the pro-angiogenic cytokines IL-8 and CXCL1. Consistent with recent TCGA findings that high-grade serous ovarian and basal-like breast cancers share many molecular similarities [11] , they both had markedly increased IL-8 and CXCL1 expression profiles in comparison with luminal breast cancers. Consistent with prior reports [15] , [17] , we found that high expression levels of IL-8 (and in some cases CXCL1 ) was strongly associated with worse outcome in ovarian, lung, renal and basal-like breast cancers. To corroborate these observations, systemic miR-200 delivery in these cancer subtypes had significant anti-angiogenic and therapeutic effects. Furthermore, we established a causal link between miR-200 regulation of IL-8 and the observed therapeutic effects. Beyond being potent pro-angiogenic cytokines, IL-8 and CXCL1 also have known roles in promoting tumour self-seeding, chemoresistance and metastasis in various models [36] , [37] . Interestingly, through several lines of evidence we found that miR-200 also has direct effects on tumour-associated endothelial cells. Although in part through IL-8 inhibition, this is likely a pleiotropic effect of several target genes (that is, CXCL1 , Ets-1 and so on). Using our well-characterized nanoparticle platforms, we demonstrated the marked therapeutic potential of miR-200 delivery into the tumour-associated endothelium, which induced vascular normalization. As angiogenesis is regulated by the balance of pro-angiogenic and anti-angiogenic factors [29] , [38] , these findings place the miR-200 family as novel, endogenous angiogenesis inhibitors. The ability of the miR-200 family to target several important cancer pathways, such as EMT and angiogenesis, is highly attractive. Although potential challenges with therapeutic RNA interference still remain, we believe the outlook of bringing therapeutic miRNA delivery to the clinic is promising [26] . The previously unrecognized role of miR-200 in angiogenesis regulation, by direct and indirect effects on tumour endothelium, substantially broadens the breadth of biologic and therapeutic implications of this miRNA family. In summary, we provide a new understanding of the role of the miR-200 family in various cancer types and provide a molecular and biological basis of divergent clinical outcomes in these cancers based on miR-200 expression. Specifically, miR-200 members can have pronounced therapeutic effects on decreasing angiogenesis and metastasis formation in ovarian, lung, renal and basal-like breast cancer models through IL-8 and CXCL1 regulation. These findings have important translational implications on the path to clinical development of miRNA-based therapies. Cell culture All cell lines were maintained in 5% CO 2 /95% air at 37 °C. Ovarian (ES2, HeyA8, SKOV3ip1, OVCAR8-ip1, A2780, A2774, IGROV1-ap1, OVCAR5), breast (MDA-MB-231, BT-549, H578T, MCF-7, T47D), renal (A498, SN12C, CAK1) and lung (H1299, H226 and A549) cancer cells were obtained from the ATCC (unless otherwise specified) and were maintained in either DMEM or RPMI 1640 (depending on cell line) supplemented with 10–15% fetal bovine serum (FBS) and 0.1% gentamicin sulphate (GeminibBioproducts, Calabasas, CA). The 344SQ (murine) and 393P (murine) cell lines were kindly provided by Dr John Kurie (MD Anderson Cancer Center, Houston, TX). RF24 endothelial cells were a kind gift of Arjan W Griffioen (VU University Medical Center, The Netherlands) and have been previously described [39] . RF24 cells were maintained in MEM supplemented with 10% FBS, sodium pyruvate, MEM vitamins, L -glutamine and MEM non-essential amino acids. 10T1/2 pericyte-like cells were maintained in basal medium Eagle with 10% FBS. All cell lines were routinely tested to confirm the absence of Mycoplasma , and all in-vitro experiments were conducted with 60–80% confluent cultures. All cells were reverse-transfected with RNAiMax reagent (Invitrogen) using pre-miR miRNA precursor molecules for miR-200a, miR-200b and negative control 1 (Ambion) at a final concentration of 20–40 nM. For miRNA inhibitor (Ambion) experiments, cells were transfected at 50 nM. Media was changed 4 h following transfections to minimize toxicity. In-vivo models and tissue processing Female athymic nude mice were purchased from the National Cancer Institute, Frederick Cancer Research and Development Center (Frederick, MD). These animals were cared for according to guidelines set forth by the American Association for Accreditation of Laboratory Animal Care and the US Public Health Service policy on Human Care and Use of Laboratory Animals. All mouse studies were approved and supervised by the MD Anderson Cancer Center Institutional Animal Care and Use Committee. All animals used were between 8 and 12 weeks of age at the time of injection. For all animal experiments, cells were trypsinized, washed and resuspended in Hanks’ balanced salt solution (HBSS; Gibco, Carlsbad, CA) before injection. For 344SQ, cells were either injected s.c. over the posterior flank (1 × 10 5 for wild-type cells, 1 × 10 6 for stable lentiviral clones in 100 μl HBSS) or by an intrapulmonary technique (5 × 10 3 in 50 μl 1:1 mixture of HBSS and BD Matrigel (BD Biosciences)) as previously described [40] . For the intrapulmonary injections, mice were anaesthetized with ketamine+xylazine and placed in the right lateral decubitus position. Following skin cleaning with an alcohol swab, an incision parallel to the rib cage between ribs 10 and 11 was made to visualize the lung through the thorax. A 1-ml tuberculin syringe with a 30-g needle was used to inject the cell suspension directly into the lung parenchyma at the left lateral dorsal axillary line. After injection, the incision was closed using surgery clips and the mice were turned on the left lateral decubitus until fully recovered. For the orthotopic ovarian models, HeyA8 (2.5 × 10 5 ) or A2774 (1 × 10 6 ) cells were injected into the peritoneal cavity. For the orthotopic breast cancer model, BT549 cells (1 × 10 6 in 50 μl 1:1 mixture of HBSS and BD Matrigel (BD Biosciences)) were injected into the fourth mammary fat pad once mice were anaesthetized with ketamine+xylazine. For the subcutaneous ovarian and renal models, HeyA8 (5 × 10 5 ) or A498 (4 × 10 6 ) cells, respectively, were injected s.c. in 100 μl HBSS. Biodistribution studies were performed to assess nanoparticle delivery of oligonucleotides. For the subcutaneous model, i.v. delivery of DOPC containing a scrambled oligonucleotide either with or without Quasar 570 (Biosearch Technologies) labelling was delivered, and at 48 h tumours were assessed. For the orthotopic lung model, 2 weeks after cell injection, nude mice were given Cy5.5-labelled oligonucleotides-DOPC (6 by i.v. and 6 by i.p. route) or unlabelled-oligonucleotide-DOPC (6 by i.v. and 6 by i.p. route). Forty-eight hours later, fluorescence imaging of excised tumour and organs was performed using the Xenogen IVIS 200 system. Cy5.5 fluorophore excitation ( λ excitation =678 nm) and emission ( λ emission =703 nm) filter sets were used. Using Living image 2.5 software, regions of interest were drawn for each organ and the total radiant efficiency (p s −1 )/(μW cm −2 ) was measured. To assess the ability to delivery miRNA into endothelial cells, Cy3-labelled control miRNA (MiR 7901, Mirus Technology) was packaged within chitosan nanoparticles and delivered i.v. into five nude tumour-bearing mice. Forty-eight hours following delivery, mice were killed and endothelial cells were assessed for colocalization of Cy3 signal. To determine optimal dosing intervals for treatment experiments, three mice bearing 344SQ subcutaneous tumours were given DOPC/miR-200b (200 μg kg −1 per mouse) i.v. and then killed at 24, 48 or 96 h. Two tumours from non-treated mice served as negative controls. Target gene modulation (ZEB1 and ZEB2) were assessed by real-time PCR, western blotting and immunohistochemistry analysis to determine the maximal effect. For all therapeutic experiments, a dose of 200 μg miRNA per kg per mouse was used. For ovarian cancer models (HeyA8 and A2774), twice weekly treatments started 1 week after cell injection and continued for ~4 weeks. For lung cancer models (344SQ), twice weekly treatments started the day following injection and continued for nearly 3 weeks. For breast cancer models (BT549), twice weekly treatments started 1 week following injection of cell lines and continued for 4 weeks. For miRNA-only experiments (HeyA8, A498, 344SQ and BT549), mice were randomly divided and treated with miRNA incorporated in neutral nanoliposomes (i.p. administration). For direct endothelial targeting (A2774), mice were randomly divided and treated with miRNA incorporated in RGD-labelled chitosan (i.v. administration) according to the following four groups ( n =10 per group): control miRNA-RGD-CH, miR-200a-RGD-CH, miR-200b-RGD-CH and miR-200a+miR-200b-RGD-CH. In all experiments, once mice in any group became moribund they were all killed, necropsied and the tumour cells were collected. Tumour weights, number and location of tumour nodules were recorded. Tumour tissue was either fixed in formalin for paraffin embedding, frozen in optimal cutting temperature (OCT) media to prepare frozen slides, or was snap-frozen for lysate preparation. Vessel permeability and structure For assessment of vessel permeability and structure, female nude mice were injected with HeyA8 ovarian cells (5 × 10 5 per mouse) into the peritoneum. Two weeks following cell injection, mice were randomly distributed to the following groups ( n =5 per group): (1) control miRNA-CH or (2) combination miR-200a+200b-CH. Twice weekly treatments were administered i.v. for a total of three serial treatments. For vessel permeability, 24 h following the third nanoparticle delivery, three mice from each group were injected with 100 μl of 10 mg ml −1 FITC-dextran (2,000,000 MW; Sigma) 1 hour before killing. Tumours were frozen in OCT and were subsequently stained with CD31. Quantification of extravascular FITC-dextran was carried out using fluorescent microscopy under the green fluorescent filter using the following scoring system: 0 points, no staining; 1 point, focal or <25%; 2 points, 25–50%, 3 points, 50–75%; 4 points, 75–100% FITC-dextran (use 8–10 sections per tumour at × 20 magnification). For vessel structure assessment, 24 h following the third nanoparticle delivery, two mice from each group were anaesthetized with isofluorane and then injected i.v. with 100 μl fluorescent-labelled Lectin (Vector Laboratories). Five minutes later, mice were perfused through the left ventricle with 4% paraformaldehyde (20 ml) for 2 min. Tumours were extracted and fixed in 4% paraformadehyde for 2 h, followed by immersion in 30% sucrose overnight, then were embedded in OCT for subsequent sectioning and visualization using confocal microscopy. Lentiviral clone generation Stable lentiviral clones expressing miR-200a, miR-200b and both miR-200a+miR-200b (miR-200ba) were generated by subcloning from a pLMP-cherry retroviral vector (kindly provided by Dr John Kurie, MD Anderson Cancer Center) expressing miR-200ba429. Oligonucleotides for miR-200a, miR-200b and miR-200ba were annealed into the lentiviral pCDH-CMV-MCS-EF1-Puro complementary DNA expression vector using the Xba I and Bam HI restriction enzymes sites. The following primer sets were used: miR-200a- Xba I-F: 5′-TGCTCTAGAGGTTCTTCCCTGGGCTTC-3′; miR-200a- Bam HI-R: 5′->CGGGATCCGAGTAGGAGCTCCGGATGTG-3′; miR-200b- Xba I-F: 5′-TGCTCTAGACAGGACCCAAAGCTGGTG-3′; miR-200b- Bam HI-R: 5′-CGGGATCCGGTCTCTGAGATGCTGGTGG-3′. XL10-gold ultracompetent cells (Stratagene, catalogue number 200314) were transformed with the annealed lentiviral vector and were grown overnight at 37 °C overnight. PCR reaction was run on a 1.2% agarose gel in 1 × TAE buffer to identify clones with the correct insert (miR-200a: 191 bp, miR-200b: 442 bp, miR-200ba: 1,062 bp, fragment of vector: 7.3 kb). The CMVF primer was sequenced to verify proper insertion. The DNA was then sequenced to test for proper insertion and cloning. The lentivirus was then produced by transfecting human embryonic kidney cells (293FT; Invitrogen) with the sequence-verified vectors, packaging plasmid (third-generation pRRE and REV) and the envelope plasmid (third-generation VSVG). Three days later, the viral supernatant was collected and filtered to remove cellular debris. Cells were transfected with each lentiviral vector (-EV, -miR-200a, -miR-200b and -miR-200ba) and selected with growth medium containing puromycin at the following concentrations (in μg ml −1 ): 344SQ, 4.0; U251, 2.0; SNB19, 0.5; ES2, 1.0; and HeyA8, 1.0. The same procedure was used to develop HeyA8 lentiviral clones expressing IL-8 shRNA or IL-8 cDNA. A validated IL-8 shRNA sequence (V2LHS_111543, accession number NM_000548, sequence: 5′-TTTGCTTGAAGTTTCACTG-3′) and the IL-8 ORF (PLOHS_100003194) was obtained from Open Biosystems before insertion and cloning. Migration assays Using modified Boyden chambers (Coster, Boston, MA) coated with 0.1% gelatin, RF24 or 10T1/2 cells (1 × 10 5 ) suspended in 100 μl serum-free media were added into the upper chamber 24 h following miRNA transfection. Complete media for RF24 containing 5% FBS (500 μl) was added to the bottom chamber as a chemo-attractant. For rescue experiments (RF24 cells), 10 ng ml −1 of recombinant human IL-8 (R&D Systems, Minneapolis, MN) was added to complete media as a chemo-attractant. The chambers were incubated at 37 °C in 5% CO 2 for 6 h. After incubation, the cells in the upper chamber were removed with cotton swabs. Migrated cells were fixed and stained, and were counted by light microscopy. Cells from five random fields were counted. Experiments were done in duplicate and performed three times. Tube formation assays Ninety-six-well plates were coated with 50 μl of BD Matrigel (BD Biosciences) and incubated at 37 °C for 10 min. RF24 cells (2 × 10 4 ) were plated onto the coated plates and incubated for 6 h at 37 °C. For indirect effects on tube formation, cells were incubated with conditioned media from HeyA8 clones (-EV, -200a and -200b). Direct effects on tube formation were assessed 24 h following transfection of RF24 cells and were grown in complete media plus 5% FBS. For rescue experiments, 10 ng ml −1 of recombinant human IL-8 (R&D Systems) was added to the wells. Experiments were performed in triplicate and repeated twice. Using an Olympus IX81 inverted microscope, five images per well were taken at × 100 magnification. The amount of nodes (defined as when at least three cells formed a single point) per image was quantified. To account for cell clumping, the highest and lowest value was removed from each group. In-vivo matrigel plug assay After transfecting HeyA8 cells with either negative control miRNA or the combination of miR-200a and miR-200b (all at 20 nM concentration), cells were exposed to serum-free media for 24 h. We then collected supernatants and centrifuged them to remove cells. As previously described [41] , we mixed the conditioned medium with phenol-red-free Matrigel (2:3 proportion, total 0.5 ml; BD Biosciences). We performed s.c. injections in mice for the three treatment groups ( n =2 per group), and VEGF (0.25 nM) served as positive control. We killed the mice after 8 days and extracted the Matrigel plug for haemoglobin content (QuantiChrom haemoglobin assay; BioAssay Systems). ELISA assays Human IL-8, CXCL1 and VEGFa protein levels were quantified by ELISA using the DuoSet Immunoassay kit (R&D Systems) according to the manufacturer’s protocol. ES2 and HeyA8 cells were transfected with 10 or 20 nM negative control miRNA, miR-200a or miR-200b in six-well plates. Media was changed 4 h following transfection, and 48 h after transfection supernatant was collected and stored at −80 °C. To assay conditioned media for tube formation assays, HeyA8 clones (-EV, -miR-200a and miR-200b) were plated in six-well plates and the supernatant was collected and stored at −80 °C 48 h later. For analysis of plasma IL-8 levels, blood (~600 μl per mouse) from five mice per group was obtained through cardiac puncture into EDTA tubes. Tubes were centrifuged at 25,000 g at 4 °C for 5 min, plasma was then obtained and stored at −80 °C until assay. The samples were assayed in triplicate or quadruplicate and data represents the mean concentration. Endothelial cell extraction After approval by the Institutional Review Board at MD Anderson Cancer Center, high-grade serous ovarian carcinomas and normal ovary samples were obtained immediately following resection. Samples were rinsed in 5 mM dithiothreitol in PBS for 20 min at room temperature, then in 10 mM EDTA in PBS and left on ice for 30 min. Samples were transferred to a small dish, a few drops of digestion cocktail (Elastase 250 μg ml −1 , collagenase A 2 mg ml −1 , DNAse 10 μg ml −1 ) was added and the tissue was minced for about 15 min. Tissue was further digested with collagenase A (1 g tissue per 10 ml) at 37 °C and shaken at 100–120 r.p.m. for 1 h. Cells were spun down at 1,000 r.p.m. for 5 min at room temperature and resuspended in 10 ml endothelial cell culture media (MEM medium, 15% FBS, 0.5% gentamycin, 10 ng ml −1 basal fibroblast growth factor, 2 mM L -glutamine, 1 mM Na Pyruvate, 1 × MEM non-essential amino acids and vitamins). The cell suspension was filtered through 500 μm, 250 um, 100 μm and finally 40 μm nylon mesh. The cells were then resuspended in 10 ml endothelial cell culture media. The cells were loaded into Ficoll tubes (15 ml) and pelleted at 1,800 r.p.m. at room temperature for 20 min. The 2–5 ml interface layered cells were collected, counted and resuspended in a PBS/BSA buffer solution at 10 7 cells per ml in a 1.5-ml eppendorf tube and placed on ice. Epithelial cells were removed by BerEP4 magnetic beads using a magnet and several rinsing steps. Finally, a double-positive selection for endothelial cells was performed using anti-CD31 and anti-CD146 antibodies by FACS sorting. Liposomal nanoparticle preparation miRNA for in-vivo intratumour delivery was incorporated into DOPC. DOPC and miRNA were mixed in the presence of excess tertiary butanol at a ratio of 1:10 (w/w) miRNA/DOPC. Tween 20 was added to the mixture in a ratio of 1:19 Tween 20:miRNA/DOPC. The mixture was vortexed, frozen in an acetone/dry ice bath and lyophilized. Before in-vivo administration, this preparation was hydrated with PBS at room temperature at a concentration of 200 μg miRNA per kg per injection. RGD-labelled chitosan nanoparticle preparation miRNA for in-vivo endothelial cell delivery was incorporated into RGD-labelled chitosan. RGD (molecular weight 719.82 Da) and chitosan (molecular weight 50–190 KDa) were conjugated by thiolation reaction using the cross-linking reagent SPDP (N-succinimidyl3-(2-pyridyldithio)-propionate). RGD–CH–NP was prepared based on ionic gelation of anionic tripolyphosphate and miRNA. Briefly, predetermined tripolyphosphate (0.25% w/v) and miRNA (1 μg μl −1 ) were added in RGD–CH solution, and the miRNA/RGD–CH–NP were spontaneously formed under constant stirring at room temperature. After incubation at 4 °C for 40 min, miRNA/RGD–CH–NP was collected by centrifugation (Thermo Biofuge, Germany) at 13,000 r.p.m. for 40 min at 4 °C. The pellet was washed by sterile water three times to isolate miRNA/RGD–CH–NP, which was stored at 4 °C until used. Immunoblotting Lysates from cultured cells were prepared using modified RIPA buffer (50 mM Tris–HCl (pH 7.4), 150 mM NaCl, 1% Triton, 0.5% deoxycholate) plus 25 μg ml −1 leupeptin, 10 μg ml −1 aprotinin, 2 mM EDTA and 1 mM sodium orthovanadate. To prepare lysates of snap-frozen tissue from mice, ~30-mm 3 cuts of tissue were disrupted with a tissue homogenizer and centrifuged at 13,000 r.p.m. for 30 min within modified RIPA buffer. The protein concentrations were determined using a BCA Protein Assay Reagent kit (Pierce Biotechnology, Rockford, IL). Lysates were loaded and separated on 8% SDS–polyacrylamide gel electrophoresis. Proteins were transferred to a nitrocellulose membrane by semidry electrophoresis (Bio-Rad Laboratories, Hercules, CA) overnight, blocked with 5% milk for 1 h and then incubated at 4 °C with primary antibody (E-cadherin (1:5,000; BD Transduction Laboratories, 610181)) overnight. After washing with TBST, the membranes were incubated with horseradish peroxidase-conjugated horse anti-mouse IgG (1:2,000; GE Healthcare, UK) for 2 h. Horseradish peroxidase was visualized by use of an enhanced chemiluminescence detection kit (Pierce). To confirm equal sample loading, the blots were probed with an antibody specific for either β-actin (0.1 μg ml −1 ; Sigma). Densitometry was calculated using ImageJ software. Quantitative real-time PCR For mRNA quantification, total RNA was isolated by using a Qiagen RNeasy kit. Using 500 ng of RNA, cDNA was synthesized by using a Verso cDNA kit (Thermo Scientific) as per the manufacturer’s instructions. Analysis of mRNA levels was performed on a 7500 Fast Real-Time PCR System (Applied Biosystems) with SYBR Green-based real-time PCR. Specific primers for (ZEB1 (murine) (forward)-5′-ATGCTCTGAACGCGCAGC-3′, (reverse)-5′-AATCGGCGATCTTTGAGAGCT-3′; ZEB2 (murine) (forward)-5′-GGAAGAGTTGATGCCACGGT-3′, (reverse)-5′-TCCGTCAAGTCACAGGGCTC-3′; IL-8 (forward)-5′-AGCACTCCTTGGCAAAACTG-3′, (reverse)-5′-CGGAAGGAACCATCTCACTG-3′; CXCL1 (human) (forward)-5′-CTTCCTCCTCCCTTCTGGTC-3′, (reverse)-5′-GAAAGCTTGCCTCAATCCTG-3′; CXCL1 (murine) (forward)-5′-GCTGGGATTCACCTCAAGAA-3′, (reverse)-5′-AAGGGAGCTTCAGGGTCAAG-3′; Ets-1 (forward)-5′-TCATTTCTTTGCTGCTTGGA-3′, (reverse)-5′-AAGCCGACTCTCACCATCAT-3′) were used; 18S rRNA was used as a housekeeping gene. PCR was done with reverse-transcribed RNA and 100 ng μl −1 of sense and antisense primers in a total volume of 20 μl. Each cycle consisted of 15 s of denaturation at 95 °C and 1 min of annealing and extension at 60 °C (40 cycles). For miRNA quantification, total RNA was isolated using Trizol (Invitrogen) extraction. TaqMan miRNA assays (Applied Biosystems) were used for reverse transcription and real-time PCR according to the manufacturer’s instructions. RNU6B was used as a housekeeping gene. Statistical analysis For animal experiments, ten mice were assigned per treatment group. This sample size gave 80% power to detect a 50% reduction in tumour weight with 95% confidence. Mouse and tumour weights and the number of tumour nodules for each group were compared using Student’s t- test (for comparisons of two groups) and analysis of variance (for multiple group comparisons). For values that were not normally distributed (as determined by the Kolmogrov–Smirnov test), the Mann–Whitney’s rank sum test was used. A P -value less than 0.05 was deemed statistically significant. All statistical tests were two-sided and were performed using SPSS version 12 for Windows statistical software (SPSS, Inc., Chicago, IL). How to cite this article: Pecot, C. V. et al. Tumour angiogenesis regulation by the miR-200 family. Nat. Commun. 4:2427 doi: 10.1038/ncomms3427 (2013).